Neuronal influence on peripheral circadian oscillators in pupalDrosophilaprothoracic glands Rhythmic expression of period ( per ) and timeless ( tim ) genes in central circadian pacemaker neurons and prothoracic gland cells, part of the peripheral circadian oscillators in flies, may synergistically control eclosion rhythms, but their oscillatory profiles remain unclear. Here we show differences and interactions between peripheral and central oscillators using per -luciferase and cytosolic Ca 2+ reporter (yellow cameleon) imaging in organotypic prothoracic gland cultures with or without the associated central nervous system. Isolated prothoracic gland cells exhibit light-insensitive synchronous per -transcriptional rhythms. In prothoracic gland cells associated with the central nervous system, however, per transcription is markedly amplified following 12-h light exposure, resulting in the manifestation of day–night rhythms in nuclear PER immunostaining levels and spontaneous Ca 2+ spiking. Unlike PER expression, nuclear TIM expression is associated with day–night cycles that are independent of the central nervous system. These results demonstrate that photoreception and synaptic signal transduction in/from the central nervous system coordinate molecular 'gears' in endocrine oscillators to generate physiological rhythms. Nearly all forms of life depend on the circadian clock system, for which transcriptional rhythms of clock genes are a common intracellular mechanism [1] , to enable temporal optimization of physiological activities and behaviours. For holometabolous insects such as Drosophila melanogaster , the timing of eclosion (emergence of the adult insect from the pupal case) is critical for survival, so pupal circadian clock genes likely regulate cellular processes underlying eclosion. Indeed, the dramatic effects of Drosophila period ( per ) mutations on the circadian rhythms of eclosion identified per as an important clock gene in flies [2] . Endocrine cells in the ring gland (RG) include both the prothoracic gland (PG) and corpus allatum (CA) cells, which release ecdysteroids and juvenile hormones, respectively [3] . PG and CA cells comprise the largest cell clusters that express the clock genes per and timeless ( tim ) in the pupae of Drosophila [4] . PG cells are considered to be circadian pacemaker cells gating eclosion timing, because when tim is over-expressed in these cells, arrhythmic eclosion occurs under conditions of constant darkness (DD) [5] . A reduction in the rhythmic release of ecdysteroids from PG cells, which depends on intracellular inositol 1,4,5-trisphosphate and Ca 2+ signalling, has been proposed as the mechanism of initiating the endocrine cascade required for eclosion [6] , [7] , [8] . Interrelations between clock gene oscillations and cellular physiological activities, however, have not been clearly characterized. Whether PG cell oscillations are solely sufficient to drive eclosion rhythms is also an unsettled question, because arrhythmic eclosion under DD has been observed in mutant flies with ablated central circadian pacemaker neurons or lateral neurons (LNs); or flies lacking pigment-dispersing factor (PDF) [5] , a neuropeptide released from LNs [9] , [10] . LN efferents terminate on a pair of neurons containing prothoracicotropic hormone that project to PG cells [11] , suggesting that PG cell oscillations are under the influence of LNs. On the other hand, circadian rhythms in nuclear translocation of per protein (PER) are resistant to the Na + channel blocker tetrodotoxin (TTX) in PG cells in RG cultures associated with the central nervous system (CNS–RG complexes) maintained under a 12-h:12-h light–dark (LD) cycle [4] . Thus, the importance of neural networks on the physiological activity of PG cells and clock-gene transcriptional oscillations in PG cells is currently obscure. It is widely accepted that the circadian clock system in animals consists of central pacemaker neurons and various peripheral oscillator cells. For example, in mammals, circadian rhythms in PER-immunoreactivity (ir) and/or per promoter-driven luciferase ( per-luc ) levels were observed not only in central pacemakers (that is, hypothalamic suprachiasmatic nucleus neurons) but also in fibroblasts [12] , the liver, lungs, and muscles [13] . Also, in flies, circadian rhythms in PER-ir and/or per-luc levels have been reported not only in LNs [14] , [15] , [16] , but also in Malpighian tubules [17] , PG cells [4] , [5] , antennae, legs and wings [18] , [19] . The discovery of molecular oscillations in various types of cells introduces de novo concepts of 'peripheral clock' or 'peripheral oscillators', and the fundamental differences between peripheral and central oscillators need to be elucidated. In mammalian fibroblasts, the amplitude of the per-luc oscillation in each cell is maintained, but synchrony is lost during the process of cell culture [20] . Thus, it has been suggested that inter-cellular communication may be the principal difference in the mechanisms underlying central and peripheral oscillators. Recently, Sellix et al . succeeded in imaging single-cell bioluminescence in dorsal LNs and large ventral LNs in Drosophila whole-brain cultures and demonstrated sustenance of tim promoter-driven luciferase rhythms in these cells [16] . In Drosophila peripheral cells, however, oscillatory profiles have not been visualized at the single-cell level. Therefore, in the present study, stable RG cultures were established, with or without the associated CNS, and circadian dynamics of per transcription, nuclear PER-/TIM-ir and cytosolic free-Ca 2+ concentrations ([Ca 2+ ] c ) in single PG cells were visualized. The results demonstrate that per -transcriptional rhythms in PG cells were phase-coupled in isolated RG cultures, and that these rhythms were amplified by CNS-dependent photoreception. Because the photic input also amplified PER-ir and Ca 2+ spiking rhythms, the dominant output from PG cells seems to depend on neural input. On the other hand, nuclear TIM-ir rhythms in PG cells were driven by local photoreception within the RG, and thus we demonstrate dissociable clock components as a profile of this endocrine oscillator. Per -transcriptional rhythms in PG cells Organotypic cultures of CNS–RG complexes or cultures of isolated RGs were established ( Fig. 1a,b ; Supplementary Fig. S1 ). To examine oscillatory gene expression profiles, a deep-cooled electron multiplier (EM) charge-coupled-device (CCD) camera was used for bioluminescence video imaging in individual PG cells from transgenic flies expressing per-luc [21] . Long-lasting circadian oscillations in per-luc expression were observed in PG cells in both CNS–RG complexes and isolated RGs ( Fig. 1c,f ; Supplementary Movies 1 and 2 ). PG cell oscillations in the CNS–RG complex were initiated in the proximal portion of the RG, which receives projections from the CNS, and the waves were propagated to the distal end ( Supplementary Fig. S2 ; Supplementary Movie 1 ). In contrast, PG cell oscillations in the isolated RG did not exhibit directional wave propagation. Oscillations in each individual PG cell, however, were synchronized ( Supplementary Movie 2 ). These results provide direct evidence for the presence of self-sustaining circadian oscillators in Drosophila endocrine cells, and demonstrate the effects of an attached CNS on the rhythms. 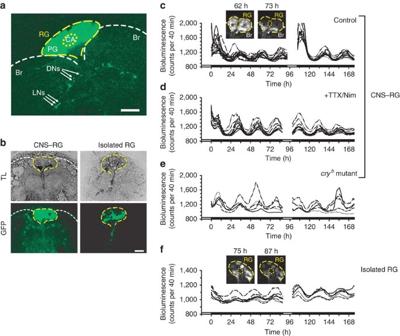Figure 1: Visualization ofper-transcriptional rhythms in single PG cellsin vitro. (a) GFP expressed in a CNS–RG complex culture from aper-luc/tim-gal4;UAS-GFPII S65T/+fly after 12 hin vitro. GFP fluorescence was concentrated between brain hemispheres (Br; white dashed lines) in the RG (yellow dashed line), which contains the PG and CA (yellow dotted line). Arrows indicate GFP-positive LNs and dorsal neurons (DNs). Scale bar, 100 μm. (b) GFP-positive cells in a CNS–RG complex culture (left) and an isolated RG (right) after 10 daysin vitro. Transmitted light (TL) images show connective tissue spread laterally from the isolated RG, but containing no GFP-positive LNs or DNs. Scale bar, 100 μm. (c)Pertranscript signal intensity changes in single PG cells in the CNS–RG complex. Different line types (for example, dashed with two dots) indicate data from a single cell. Oscillations were of high amplitude at the beginning of recordings, which rapidly reduced under DD. Data from four different cultures were superimposed. One organotypic culture re-exposed to 12 h of light (120 lux) exhibited a similar transition at the beginning of recording. (d) A similar experiment, but CNS–RG complexes were cultured in medium containing TTX (0.3 μM) and nimodipine (Nim; 2 μM). The light-to-dark transition response was blocked. (e) A similar experiment, but CNS–RG complexes were cultured fromcrybmutants. The light-to-dark transition response was blocked. (f)Pertranscript signal intensity changes in single PG cells in isolated RG cultures of wild-type flies. Steady low-amplitude circadian oscillations were observed with no light-to-dark transition. Smaller absolutepertranscript signal in isolated RGs compared with CNS–RG complexes. All the above bioluminescence measurements were conducted in culture medium containing 1 mM luciferin, without any medium exchange during the entire recording period. White and black bars on the bottom indicate light and dark periods, respectively. Images in (c) and (f) indicate example bioluminescence images collected at the circadian peak and trough. The corresponding GFP images at the end of the experiments are shown in (b). Figure 1: Visualization of per -transcriptional rhythms in single PG cells in vitro . ( a ) GFP expressed in a CNS–RG complex culture from a per-luc/tim-gal4 ; UAS-GFPII S65T/+ fly after 12 h in vitro . GFP fluorescence was concentrated between brain hemispheres (Br; white dashed lines) in the RG (yellow dashed line), which contains the PG and CA (yellow dotted line). Arrows indicate GFP-positive LNs and dorsal neurons (DNs). Scale bar, 100 μm. ( b ) GFP-positive cells in a CNS–RG complex culture ( left ) and an isolated RG ( right ) after 10 days in vitro . Transmitted light (TL) images show connective tissue spread laterally from the isolated RG, but containing no GFP-positive LNs or DNs. Scale bar, 100 μm. ( c ) Per transcript signal intensity changes in single PG cells in the CNS–RG complex. Different line types (for example, dashed with two dots) indicate data from a single cell. Oscillations were of high amplitude at the beginning of recordings, which rapidly reduced under DD. Data from four different cultures were superimposed. One organotypic culture re-exposed to 12 h of light (120 lux) exhibited a similar transition at the beginning of recording. ( d ) A similar experiment, but CNS–RG complexes were cultured in medium containing TTX (0.3 μM) and nimodipine (Nim; 2 μM). The light-to-dark transition response was blocked. ( e ) A similar experiment, but CNS–RG complexes were cultured from cry b mutants. The light-to-dark transition response was blocked. ( f ) Per transcript signal intensity changes in single PG cells in isolated RG cultures of wild-type flies. Steady low-amplitude circadian oscillations were observed with no light-to-dark transition. Smaller absolute per transcript signal in isolated RGs compared with CNS–RG complexes. All the above bioluminescence measurements were conducted in culture medium containing 1 mM luciferin, without any medium exchange during the entire recording period. White and black bars on the bottom indicate light and dark periods, respectively. Images in ( c ) and ( f ) indicate example bioluminescence images collected at the circadian peak and trough. The corresponding GFP images at the end of the experiments are shown in ( b ). Full size image Moreover, when the CNS–RG complex was transferred from LD to DD, we observed a high amplitude per transcription signal for one 12-h cycle, then an immediate reduction in amplitude for the remaining time under DD ( Fig. 1c ). This LD-to-DD transition response was blocked with the removal of synaptic input from the CNS, either pharmacologically with TTX (0.3 μM) and the L-type Ca 2+ channel inhibitor nimodipine (2 μM; Fig. 1d ) or by physical isolation of the RG from the CNS ( Fig. 1f ). In addition, the LD-to-DD transition response was blocked in the CNS–RG complexes cultured from cry b mutants, which contain a loss-of-function mutation for the circadian photoreceptor cryptochrome (CRY) [22] , [23] ( Fig. 1e ). The LD-to-DD response was reproducible in the CNS–RG complex, when the cultures were re-exposed to 12 h of light ( Fig. 1c ; Supplementary Fig. S3 ). Thus, this transition response seems to depend on prior photic input to the CNS–RG complex. The subsequent reduced-amplitude expression in the CNS–RG complex maintained for several days under DD was similar to that observed in the isolated RG. Aside from the beginning of the recordings in the CNS–RG complex, the phase of each PG cell oscillation was highly synchronized. These results demonstrate that intrinsic PG cell oscillations in per transcription are of much smaller amplitude than those in PG cells receiving photic signals via the CNS. To further characterize the oscillatory response of per-luc to light, the CNS–RG complex was exposed to a brief (30-min) light pulse ( Fig. 2 ). The light pulse did not amplify the per-luc oscillations, but produced phase delays or advances, depending on the time of exposure. For example, a light-pulse immediately after the peak in per-luc rhythms produced advance-shifts in successive rhythms ( Fig. 2a , left), whereas light-pulses, immediately before the peak of per-luc rhythms, produced delay-shifts in successive rhythms ( Fig. 2a , right). Because a single CNS–RG complex contains multiple PG cells that oscillate in slightly different phases, light-pulses applied in the approximate middle of the peak of the tissue-averaged per-luc rhythm, produced bi-directional phase-shifts and de-synchronized each individual PG cell rhythm, resulting in a significant reduction in the average oscillation amplitude ( Fig. 2b ). A significant reduction in the averaged amplitude following a light pulse exposure at a critical circadian time corresponds to loss of eclosion rhythms under similar circumstances [24] . This phenomenon termed 'singularity' has been modelled using Per2-luciferase rhythms in mammalian fibroblasts overexpressing melanopsin as an artificial photoreceptor [25] . To our knowledge, however, the present results are the first demonstration of the cellular singularity-like behaviours in multicellular organs. The photic information underlying the phase-shifts is presumably processed in the CNS, because isolation of RG or treatment with TTX and nimodipine for the CNS–RG complex blocked the light-induced phase-shifts ( Fig. 2a ). Also, CRY may have a pivotal role in the photoreception in the CNS, because PG cells cultured from cry b flies exhibited significantly smaller phase-responses, consistent with the eclosion rhythm profiles in cry b flies [26] . Most importantly, the phase-response curve, obtained from these cellular events ( Fig. 2c ), was well matched to the light-induced phase-response curve for Drosophila eclosion rhythms [27] , suggesting that oscillatory outputs from PG cells may determine the timing of eclosion in flies. 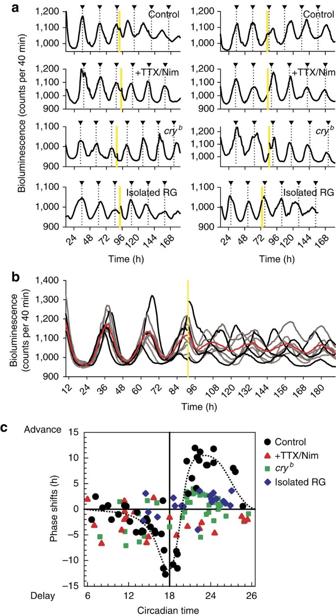Figure 2: Light-pulse-induced circadian phase-shifts of single PG cells in the CNS–RG complex. (a) Each trace denotes a representativeper-lucrhythm in a single PG cell that received a 30-min light-pulse (yellow bar) immediately after (left) or before (right) the peak ofper-lucrhythms. Triangles on the top denote the peak ofper-lucrhythms estimated by the waveforms before light-pulse exposure and extended to the end of recordings as a reference. First row: in PG cells in CNS–RG complex cultures, a light-pulse immediately after the peak produced phase-advance and a light-pulse immediately before the peak produced phase-delay in successiveper-lucrhythms. Second row: an experiment similar to the above, but CNS–RG complexes were cultured in medium containing TTX (0.3 μM) and nimodipine (Nim; 2 μM). Light-induced phase-advance and -delay were both blocked by TTX and Nim. Third row: an experiment similar to the above, but CNS–RG complexes were cultured fromcrybmutant flies. Light-induced phase-shifts were significantly reduced in thecrybmutant. Bottom row: in PG cells in isolated RG cultures from wild-type flies, light-pulse-induced phase-shifts were significantly reduced. (b) Synchronousper-lucrhythms in individual PG cells (grey-scale traces) located in a CNS–RG complex were desynchronized by a 30-min light-pulse given at the approximate middle of the peak ofper-lucrhythms. The average amplitude ofper-lucrhythms (red trace) was significantly reduced after the light-pulse. (c) Circadian time dependency of light-induced phase-shifts ofper-lucrhythms in PG cells. Circadian time 18 was defined by the peak ofper-lucrhythms during the pre-exposure period. The second circadian peak after the light pulse was used to estimate phase-shifts. Under control conditions (black circles), light-pulses produced a phase-response curve (hand-fitted curve as dotted line) in which delay shifts switched to advance shifts at circadian time 20. The light-induced phase-responses were reduced by TTX/Nim treatment (red triangles), in PG cells cultured fromcrybmutant flies (green squares) and in PG cells from isolated RG cultures (blue diamonds). Figure 2: Light-pulse-induced circadian phase-shifts of single PG cells in the CNS–RG complex. ( a ) Each trace denotes a representative per-luc rhythm in a single PG cell that received a 30-min light-pulse (yellow bar) immediately after ( left ) or before ( right ) the peak of per-luc rhythms. Triangles on the top denote the peak of per-luc rhythms estimated by the waveforms before light-pulse exposure and extended to the end of recordings as a reference. First row: in PG cells in CNS–RG complex cultures, a light-pulse immediately after the peak produced phase-advance and a light-pulse immediately before the peak produced phase-delay in successive per-luc rhythms. Second row: an experiment similar to the above, but CNS–RG complexes were cultured in medium containing TTX (0.3 μM) and nimodipine (Nim; 2 μM). Light-induced phase-advance and -delay were both blocked by TTX and Nim. Third row: an experiment similar to the above, but CNS–RG complexes were cultured from cry b mutant flies. Light-induced phase-shifts were significantly reduced in the cry b mutant. Bottom row: in PG cells in isolated RG cultures from wild-type flies, light-pulse-induced phase-shifts were significantly reduced. ( b ) Synchronous per-luc rhythms in individual PG cells (grey-scale traces) located in a CNS–RG complex were desynchronized by a 30-min light-pulse given at the approximate middle of the peak of per-luc rhythms. The average amplitude of per-luc rhythms (red trace) was significantly reduced after the light-pulse. ( c ) Circadian time dependency of light-induced phase-shifts of per-luc rhythms in PG cells. Circadian time 18 was defined by the peak of per-luc rhythms during the pre-exposure period. The second circadian peak after the light pulse was used to estimate phase-shifts. Under control conditions (black circles), light-pulses produced a phase-response curve (hand-fitted curve as dotted line) in which delay shifts switched to advance shifts at circadian time 20. The light-induced phase-responses were reduced by TTX/Nim treatment (red triangles), in PG cells cultured from cry b mutant flies (green squares) and in PG cells from isolated RG cultures (blue diamonds). Full size image To carefully compare the differences in oscillatory profiles of peripheral cells, we also analysed per-luc rhythms in Malpighian tubule cultures and observed that per-luc rhythms in isolated Malpighian tubules were photoresponsive ( Supplementary Fig. S4 ). Thus, we suggest that photosensitivity of peripheral cells may depend on the cell and tissue type. Because transcriptional levels of cry were smaller in the RG compared with the brain or Malpighian tubules ( Supplementary Fig. S5 ), tissue-specific photosensitivity may be mediated by the density of CRY in each tissue. Post-transcriptional rhythms in PG cells To examine post-transcriptional rhythms in PG cells, we also analysed nuclear PER-/TIM-ir in organotypic cultures. When CNS–RG complexes were cultured under 12-h:12-h LD cycles, there was a rhythmic nuclear PER-ir in PG cells lasting 5–6 days in vitr o ( Fig. 3a ), consistent with previous observations of PER-ir in PG cells in vitro [4] and in vivo [5] . Circadian rhythms in nuclear PER-ir, however, were below the detection limit in CNS–RG complex cultures maintained under DD ( Fig. 3a ). Circadian rhythms in nuclear PER-ir were evident in cultured LNs under DD ( Fig. 3b ); thus, it appears that in DD, the autonomous outputs from central pacemaker neurons were insufficient to manifest nuclear PER-ir rhythms in PG cells. Results from the present study further demonstrate that circadian rhythms in nuclear PER-ir were below the detection limit in PG cells physically isolated from the CNS, regardless of the lighting schedule ( Fig. 3a ). These data indicate that photoreception in the CNS, signal transduction to the RG, and amplification in the gene transcriptional rhythms ( Fig. 1c ) were required for the manifestation of nuclear PER-ir rhythms in PG cells. 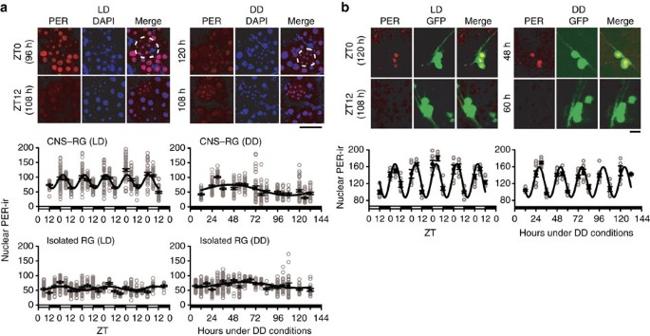Figure 3: Nuclear PER immunostaining in cultured PG cells. (a) Images: comparison of anti-PER immunoreactivity (PER-ir) in CNS–RG complexes maintained under 12-h:12-h LD or DD. The time (h)in vitrois indicated on the left. Most PER-ir (red) co-localized with DAPI (blue) nuclear staining at lights-on (ZT0; merged image was purple), but not at lights-off (ZT12), indicated by the diffuse non-nuclear red at ZT12. Cells with small nuclei (<7–8 μm) are CA cells (white dotted line) and cells with larger nuclei (>10 μm) are PG cells. No circadian rhythms in nuclear PER-ir were evident in CNS–RG cultures maintained under DD. Scale bar, 50 μm. Graphs: nuclear PER-ir in PG cells was calculated as the PER-ir/DAPI fluorescence intensity ratio at each time point. Grey circles indicate the level of nuclear PER-ir in each cell (number of cultures, 152; number of cells, 3,173). Nonlinear regression fit a sine wave to the data (solid lines). Robust circadian oscillation of nuclear PER-ir accumulation occurred only in CNS–RG complexes maintained under LD conditions (estimated period, 23.6 h), while non-circadian oscillations occurred in CNS–RG complexes maintained under DD (128.7 h) and in isolated RGs maintained under LD (52.1 h) or DD (122.6 h) conditions. (b) PER-ir in LNs in CNS–RG complex cultures. Images: high levels of PER-ir (red) were observed in LN nuclei at lights-on (ZT0) under LD conditions and during the subjective daytime (48 h under DD conditions). LNs were identified by their expression of GFP inPdf-gal4/UAS-GFPII S65Tflies. Red PER-ir and green GFP image-overlays identified LNs that exhibited rhythmic nuclear PER-ir (yellow in the merge images). Scale bar, 5 μm. Graphs: nuclear PER-ir rhythms under LD cycles exhibited an estimated period of 23.5 h. Free-running nuclear PER-ir rhythms exhibited an estimated period of 24.2 h under DD conditions. In both cases, nuclear PER-ir rhythms were sustained for five circadian cyclesin vitro. Nuclear PER-ir in LNs was calculated as the ratio of PER-ir over averaged background fluorescence intensity. Figure 3: Nuclear PER immunostaining in cultured PG cells. ( a ) Images: comparison of anti-PER immunoreactivity (PER-ir) in CNS–RG complexes maintained under 12-h:12-h LD or DD. The time (h) in vitro is indicated on the left. Most PER-ir (red) co-localized with DAPI (blue) nuclear staining at lights-on (ZT0; merged image was purple), but not at lights-off (ZT12), indicated by the diffuse non-nuclear red at ZT12. Cells with small nuclei (<7–8 μm) are CA cells (white dotted line) and cells with larger nuclei (>10 μm) are PG cells. No circadian rhythms in nuclear PER-ir were evident in CNS–RG cultures maintained under DD. Scale bar, 50 μm. Graphs: nuclear PER-ir in PG cells was calculated as the PER-ir/DAPI fluorescence intensity ratio at each time point. Grey circles indicate the level of nuclear PER-ir in each cell (number of cultures, 152; number of cells, 3,173). Nonlinear regression fit a sine wave to the data (solid lines). Robust circadian oscillation of nuclear PER-ir accumulation occurred only in CNS–RG complexes maintained under LD conditions (estimated period, 23.6 h), while non-circadian oscillations occurred in CNS–RG complexes maintained under DD (128.7 h) and in isolated RGs maintained under LD (52.1 h) or DD (122.6 h) conditions. ( b ) PER-ir in LNs in CNS–RG complex cultures. Images: high levels of PER-ir (red) were observed in LN nuclei at lights-on (ZT0) under LD conditions and during the subjective daytime (48 h under DD conditions). LNs were identified by their expression of GFP in Pdf-gal4/UAS-GFPII S65T flies. Red PER-ir and green GFP image-overlays identified LNs that exhibited rhythmic nuclear PER-ir (yellow in the merge images). Scale bar, 5 μm. Graphs: nuclear PER-ir rhythms under LD cycles exhibited an estimated period of 23.5 h. Free-running nuclear PER-ir rhythms exhibited an estimated period of 24.2 h under DD conditions. In both cases, nuclear PER-ir rhythms were sustained for five circadian cycles in vitro . Nuclear PER-ir in LNs was calculated as the ratio of PER-ir over averaged background fluorescence intensity. Full size image Robust rhythms in TIM-ir, but not in PER-ir, levels were reported for PG cells in pupae maintained for 2 days in the dark [5] . Therefore, we further quantified nuclear TIM-ir in our cultures. Interestingly, unlike PER-ir, nuclear TIM-ir rhythms in PG cells were sustained in CNS–RG complex cultures maintained under DD ( Fig. 4a ). In addition, nuclear TIM-ir rhythms in PG cells were sustained in isolated RG cultures maintained under DD. Most intriguingly, nuclear TIM-ir rhythms in PG cells entrained to LD cycles in isolated RG cultures with a peak at the end of the dark period, and CRY enrolled the LD entrainment within the RG as the peak drifted to the middle of the light period in isolated RG cultures from cry b flies ( Figs 4a and 5a ). Because per - luc rhythms neither respond to light ( Figs 1 and 2 ) nor entrain to LD cycles in the isolated RG ( Fig. 5b ), this represents differential light-input pathways for PG cell molecular gears: per transcription and translation are CNS-dependent, whereas those of tim may not be. 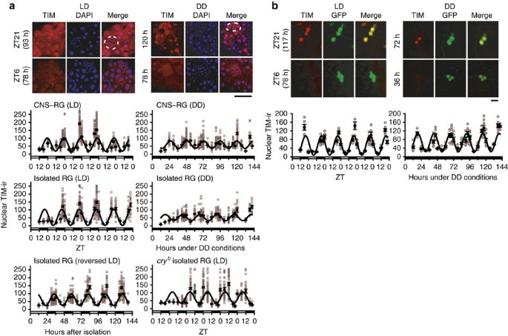Figure 4: Nuclear TIM immunostaining in cultured PG cells. (a) Images: comparison of anti-TIM-ir in CNS–RG complexes maintained under 12-h:12-h LD cycles or DD conditions. Unlike the PER-ir, nuclear TIM-ir exhibited apparent circadian rhythms in CNS–RG cultures maintained under DD. Scale bar, 50 μm. Graphs: nuclear TIM-ir in PG cells was calculated as the TIM-ir/DAPI fluorescence intensity ratio at each time point (number of cultures, 267; number of cells, 6,502). Robust circadian oscillation of nuclear TIM-ir accumulation occurred in CNS–RG complexes maintained under LD conditions (estimated period, 23.6 h) and under DD (23.5 h). Also, circadian oscillations were found in isolated RGs maintained under LD (24.4 h) or DD (24.4 h) conditions. The TIM-ir rhythms in the isolated RG entrain to LD cycles; synchronous rhythms (24.1 h) were present under reversed LD cycle conditions. CRY in the RG is essential for LD entrainment of, but not for the generation of TIM-ir rhythms in PG cells because detrained rhythms (24.8 h) were present in isolated RG cultures fromcrybmutants. (b) TIM-ir in LNs in CNS–RG complex cultures. Images: high levels of TIM-ir (red) were observed in LN nuclei in the middle of the night (ZT21) under LD conditions and in the middle of subjective night (72 h under DD conditions). LNs were identified by their expression of GFP inPdf-gal4/UAS-GFPII S65Tflies. Red TIM-ir and green GFP image-overlays identified LNs that exhibited rhythmic nuclear TIM-ir (yellow in the merge images). Scale bar, 5 μm. Graphs: day–night nuclear TIM-ir rhythms exhibited an estimated period of 23.9 h. Free-running nuclear TIM-ir rhythms exhibited an estimated period of 24.2 h under DD conditions. In both cases, nuclear TIM-ir rhythms were sustained for five circadian cyclesin vitro. Figure 4: Nuclear TIM immunostaining in cultured PG cells. ( a ) Images: comparison of anti-TIM-ir in CNS–RG complexes maintained under 12-h:12-h LD cycles or DD conditions. Unlike the PER-ir, nuclear TIM-ir exhibited apparent circadian rhythms in CNS–RG cultures maintained under DD. Scale bar, 50 μm. Graphs: nuclear TIM-ir in PG cells was calculated as the TIM-ir/DAPI fluorescence intensity ratio at each time point (number of cultures, 267; number of cells, 6,502). Robust circadian oscillation of nuclear TIM-ir accumulation occurred in CNS–RG complexes maintained under LD conditions (estimated period, 23.6 h) and under DD (23.5 h). Also, circadian oscillations were found in isolated RGs maintained under LD (24.4 h) or DD (24.4 h) conditions. The TIM-ir rhythms in the isolated RG entrain to LD cycles; synchronous rhythms (24.1 h) were present under reversed LD cycle conditions. CRY in the RG is essential for LD entrainment of, but not for the generation of TIM-ir rhythms in PG cells because detrained rhythms (24.8 h) were present in isolated RG cultures from cry b mutants. ( b ) TIM-ir in LNs in CNS–RG complex cultures. Images: high levels of TIM-ir (red) were observed in LN nuclei in the middle of the night (ZT21) under LD conditions and in the middle of subjective night (72 h under DD conditions). LNs were identified by their expression of GFP in Pdf-gal4/UAS-GFPII S65T flies. Red TIM-ir and green GFP image-overlays identified LNs that exhibited rhythmic nuclear TIM-ir (yellow in the merge images). Scale bar, 5 μm. Graphs: day–night nuclear TIM-ir rhythms exhibited an estimated period of 23.9 h. Free-running nuclear TIM-ir rhythms exhibited an estimated period of 24.2 h under DD conditions. In both cases, nuclear TIM-ir rhythms were sustained for five circadian cycles in vitro . 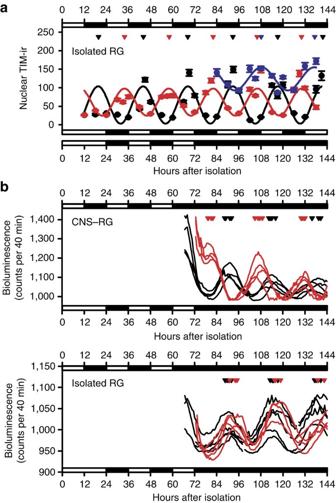Figure 5: Selective entrainment of nuclear TIM expression rhythms to LD cycles in PG cells in isolated RGs. (a) Nuclear TIM-ir rhythms in PG cells in isolated RG cultures maintained under standard LD cycles (black circles), reversed LD cycles (red circles), and DD following the reversed LD cycles (blue circles). Peak TIM-ir rhythms are marked on the top by triangles in corresponding colours. TIM-ir rhythms in PG cells were synchronized to the LD cycles in the isolated RG and had free-run under DD with an initial circadian phase coupled to the precedent LD cycles. (b) Representativeper-lucrhythms in PG cells, which was cultured under standard LD cycle conditions (black traces) or under reversed LD cycle conditions (red traces) before recordings under DD conditions. Peak ofper-lucrhythms estimated in PG cells pre-cultured under standard LD cycle conditions (black triangles) and under reversed LD cycle conditions (red triangles) were marked on the top.Per-lucrhythms in PG cells synchronized to the LD cycles in the CNS–RG complex but not in the isolated RG. Full size image Figure 5: Selective entrainment of nuclear TIM expression rhythms to LD cycles in PG cells in isolated RGs. ( a ) Nuclear TIM-ir rhythms in PG cells in isolated RG cultures maintained under standard LD cycles (black circles), reversed LD cycles (red circles), and DD following the reversed LD cycles (blue circles). Peak TIM-ir rhythms are marked on the top by triangles in corresponding colours. TIM-ir rhythms in PG cells were synchronized to the LD cycles in the isolated RG and had free-run under DD with an initial circadian phase coupled to the precedent LD cycles. ( b ) Representative per-luc rhythms in PG cells, which was cultured under standard LD cycle conditions (black traces) or under reversed LD cycle conditions (red traces) before recordings under DD conditions. Peak of per-luc rhythms estimated in PG cells pre-cultured under standard LD cycle conditions (black triangles) and under reversed LD cycle conditions (red triangles) were marked on the top. Per-luc rhythms in PG cells synchronized to the LD cycles in the CNS–RG complex but not in the isolated RG. Full size image Physiological photoresponses in PG cells Using tim-gal4/UAS-cameleon ( YC2.1-82 ) flies [28] , we also monitored [Ca 2+ ] c in cultured PG cells. PG cells in CNS–RG complex cultures exhibited spontaneous Ca 2+ spikes with periods on the order of minutes ( Fig. 6 ). The Ca 2+ spikes were resistant to the depletion of internal Ca 2+ stores with exposure to thapsigargin (1 μM; Fig. 6a ; Supplementary Fig. S6a ), but were highly sensitive to the concentration of extracellular Ca 2+ ( Fig. 6a ). Baseline [Ca 2+ ] c levels and Ca 2+ spike frequencies increased when the extracellular Ca 2+ concentration was switched back from a Ca 2+ -free buffer ( Fig. 6a ), but the store-operated Ca 2+ channel blocker SKF96365 (50 μM) had no apparent effect on this rebound response ( Supplementary Fig. S6b ). TTX (0.3 μM) transiently reduced the Ca 2+ spiking frequency, but the continued presence of TTX (0.3 μM) in the culture medium had little effect on the Ca 2+ spiking frequency ( Fig. 6b ). When the L-type Ca 2+ channel activator BayK8644 (100 μM) was applied during exposure to TTX, the Ca 2+ spiking frequency returned to baseline levels ( Fig. 6b ). Consistent with this, nimodipine (2 μM) reduced the Ca 2+ spiking frequency in PG cells cultured in TTX-supplemented medium ( Fig. 6c ). These results suggest that membrane depolarization and Ca 2+ influx through voltage-dependent Ca 2+ channels evoked Ca 2+ spikes in PG cells. 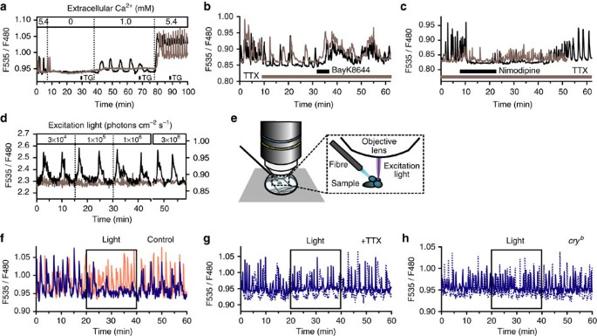Figure 6: Calcium dynamics in PG cells. The CNS–RG complexes (a–candf–h) and isolated RG (d) were cultured fromtim-gal4/UAS-cameleon(YC2.1-82) flies. Representative data from two different cells were plotted for each experiment. (a) The frequency of spontaneous Ca2+spikes depended on the extracellular Ca2+concentrations. In contrast, exposure to the Ca2+-ATPase inhibitor thapsigargin (TG; 1 min, 1 μM) had no effect on the frequency of Ca2+spikes. (b) Effects of TTX (0.3 μM) and the L-type Ca2+channel activator BayK8644 (100 μM) on Ca2+spikes in PG cells. TTX reduced the frequency but did not abolish Ca2+spikes. Exposure to BayK8644 increased the Ca2+spiking frequency again, even in the presence of TTX. (c) PG cells in CNS–RG complexes cultured in medium containing TTX exhibited Ca2+spikes similar to control culture conditions. Nimodipine (2 μM) reduced the Ca2+spiking frequency in PG cells cultured with TTX. (d) The effect of excitation light on [Ca2+]cwas tested in PG cells in isolated RG cultures using an LED light source. The low-fluorescent signals were amplified using an EM–CCD gain. The relatively noisy traces at 3×104photons cm−2s−1(invisible to eye) were caused by the electrical amplification of the signals. Neither the frequency of Ca2+spikes nor baseline [Ca2+]clevels were affected by excitation light in PG cells in isolated RG cultures. (e) To examine the effects of photic stimulation on Ca2+spikes (f–h), a micro-light was located near the brain hemisphere. An excitation light for Ca2+imaging (435–445 nm) was tightly focussed on the RG. (f) Exposure of the brain to blue (455–505 nm; blue trace) but not red (595–645 nm; red trace) light temporarily blocked Ca2+spikes in PG cells in CNS–RG complex cultures. The effects of blue light exposure (in two representative cells as solid and dashed lines) were abolished in PG cells cultured with TTX (g) or in PG cells cultured fromcrybbackground flies (h). All the above results were consistently observed in 44–119 cells in 3–5 organs. Figure 6: Calcium dynamics in PG cells. The CNS–RG complexes ( a – c and f – h ) and isolated RG ( d ) were cultured from tim-gal4/UAS-cameleon ( YC2.1-82 ) flies. Representative data from two different cells were plotted for each experiment. ( a ) The frequency of spontaneous Ca 2+ spikes depended on the extracellular Ca 2+ concentrations. In contrast, exposure to the Ca 2+ -ATPase inhibitor thapsigargin (TG; 1 min, 1 μM) had no effect on the frequency of Ca 2+ spikes. ( b ) Effects of TTX (0.3 μM) and the L-type Ca 2+ channel activator BayK8644 (100 μM) on Ca 2+ spikes in PG cells. TTX reduced the frequency but did not abolish Ca 2+ spikes. Exposure to BayK8644 increased the Ca 2+ spiking frequency again, even in the presence of TTX. ( c ) PG cells in CNS–RG complexes cultured in medium containing TTX exhibited Ca 2+ spikes similar to control culture conditions. Nimodipine (2 μM) reduced the Ca 2+ spiking frequency in PG cells cultured with TTX. ( d ) The effect of excitation light on [Ca 2+ ] c was tested in PG cells in isolated RG cultures using an LED light source. The low-fluorescent signals were amplified using an EM–CCD gain. The relatively noisy traces at 3×10 4 photons cm −2 s −1 (invisible to eye) were caused by the electrical amplification of the signals. Neither the frequency of Ca 2+ spikes nor baseline [Ca 2+ ] c levels were affected by excitation light in PG cells in isolated RG cultures. ( e ) To examine the effects of photic stimulation on Ca 2+ spikes ( f – h ), a micro-light was located near the brain hemisphere. An excitation light for Ca 2+ imaging (435–445 nm) was tightly focussed on the RG. ( f ) Exposure of the brain to blue (455–505 nm; blue trace) but not red (595–645 nm; red trace) light temporarily blocked Ca 2+ spikes in PG cells in CNS–RG complex cultures. The effects of blue light exposure (in two representative cells as solid and dashed lines) were abolished in PG cells cultured with TTX ( g ) or in PG cells cultured from cry b background flies ( h ). All the above results were consistently observed in 44–119 cells in 3–5 organs. Full size image Frequency of Ca 2+ spikes in PG cells in isolated RG cultures did not depend on the intensity of blue-violet (435–445 nm) light ( Fig. 6d ). Therefore, effects of photic signal inputs on Ca 2+ spikes in PG cells were further analysed by exposing the CNS to light ( Fig. 6e ). Exposure of the CNS to 20 min of blue (455–505 nm) light significantly reduced (−12.8±5.0%) the Ca 2+ spiking frequency (mean frequency=0.014±0.001 Hz before blue light exposure and 0.012±0.001 Hz during blue light exposure; number of cells=110 in 5 organs; P <0.05, a paired t -test; Fig. 6f ), whereas exposure to red (595–645 nm) light had small effects (mean frequency=0.013±0.001 Hz before red light exposure and 0.012±0.001 Hz during red light exposure; number of cells=44 in 3 organs, NS; Fig. 6f ). The effects of blue light exposure were abolished in CNS–RG complex cultures in TTX supplemented medium (mean frequency=0.014±0.001 Hz before blue light exposure and 0.015±0.001 Hz during blue light exposure, number of cells=119 in 5 organs, NS; Fig. 6g ). Also, PG cells in the CNS–RG complex cultured from cry b background flies overall exhibited higher Ca 2+ spike frequency (mean frequency=0.017±0.001 Hz during the entire session; number of cells=55 in 3 organs; P <0.01 in comparison with the control cry + cells, a paired t -test) and blue light exposure only partially reduced spike frequencies (−8.2±10.5%, NS; Fig. 6h ). These results indicate that CRY-dependent photoreception in the CNS inhibited PG cell activity via efferent neuronal networks. Circadian [Ca 2+ ] c dynamics in PG cells Finally, 4-point-samples were collected within 24 h to examine the effects of day–night lighting schedules on [Ca 2+ ] c in PG cells ( Fig. 7 ). PG cells in CNS–RG complex cultures exhibited robust daily rhythms in Ca 2+ spiking frequency (number of cells=130 in 6 organs): fast fourier transformation (FFT) power average in the middle of the night (zeitgeber time; ZT18) was 26% larger than that in the middle of the day (ZT6; Fig. 7a,b ). The Ca 2+ spiking frequency was reduced and the day–night variations were diminished when PG cells in CNS–RG complexes were cultured with TTX and nimodipine (number of cells=140 in 6 organs; FFT power average at ZT18 was 12% larger than that at ZT6). In addition, the Ca 2+ spiking frequency measured in PG cells in isolated RG cultures was markedly lower regardless of the time of day (number of cells=144 in 5 organs; FFT power average at ZT18 was 58% that in control cultures). These results indicate that Na + and Ca 2+ channel-dependent CNS activities contribute significantly to the generation of Ca 2+ spiking rhythms in PG cells. 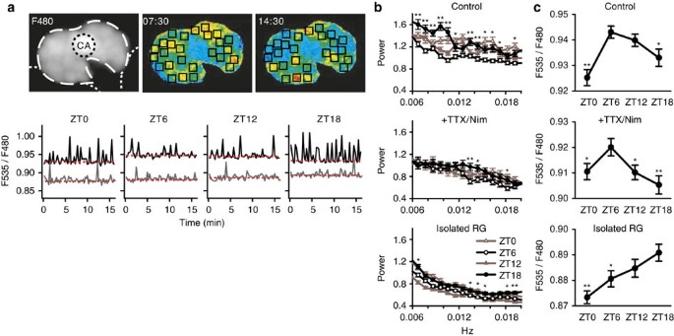Figure 7: Day–night variations in Ca2+spiking profiles in PG cells. (a) Upper left panel: An example fluorescence image (F480 nm) of a CNS–RG complex cultured from atim-gal4/UAS-cameleon(YC2.1-82) fly. The RG is indicated by the white dashed line, the CA by the black dotted line, and the CNS by the white dotted lines. Upper centre and right panels: Two virtual-colour images at different time points indicating [Ca2+]cbased on the fluorescence ratio (F535/F480 nm). Warmer colours indicate higher [Ca2+]c. Squares in the virtual-colour images indicate the approximate locations of PG cells, which exhibited Ca2+spiking with periods of ~1–3 min (0.006–0.017 Hz). The CNS in this field exhibited no fluorescence and CA cells exhibited little or no [Ca2+]coscillations. Lower panel: typical [Ca2+]coscillations in PG cells at 4 different ZTs. Each trace indicates the [Ca2+]cin a single PG cell in either CNS–RG complex (black) or isolated RG (grey) culture. The estimated baseline levels are indicated by red dotted lines. The frequency of spontaneous Ca2+spikes depended on the ZT, which was highest in the middle of the night (ZT18) in PG cells in the CNS–RG complex. (b) The Ca2+spiking frequencies in PG cells were determined using FFT analysis. In untreated CNS–RG complexes, the wide-band frequency power was higher at ZT18 than at ZT6. The overall frequency power and day–night differences were diminished in CNS–RG complexes cultured with TTX and nimodipine (+TTX/Nim) and in isolated RG cultures. *P<0.05, **P<0.01 significantly larger than the corresponding ZT6 groups, repeated one-way ANOVA followed by a Duncan's multiple range test. (c) The baseline [Ca2+]clevels in PG cells exhibited day–night variations. The highest baseline values were found at ZT6 in untreated CNS–RG complex cultures (control) and CNS–RG complexes cultured with TTX/Nim. The peak baseline value was shifted to ZT18 in isolated RG cultures. *P<0.05, **P<0.01, one-way ANOVA followed by a Duncan's multiple range test. Figure 7: Day–night variations in Ca 2+ spiking profiles in PG cells. ( a ) Upper left panel: An example fluorescence image (F480 nm) of a CNS–RG complex cultured from a tim-gal4/UAS-cameleon ( YC2.1-82 ) fly. The RG is indicated by the white dashed line, the CA by the black dotted line, and the CNS by the white dotted lines. Upper centre and right panels: Two virtual-colour images at different time points indicating [Ca 2+ ] c based on the fluorescence ratio (F535/F480 nm). Warmer colours indicate higher [Ca 2+ ] c . Squares in the virtual-colour images indicate the approximate locations of PG cells, which exhibited Ca 2+ spiking with periods of ~1–3 min (0.006–0.017 Hz). The CNS in this field exhibited no fluorescence and CA cells exhibited little or no [Ca 2+ ] c oscillations. Lower panel: typical [Ca 2+ ] c oscillations in PG cells at 4 different ZTs. Each trace indicates the [Ca 2+ ] c in a single PG cell in either CNS–RG complex (black) or isolated RG (grey) culture. The estimated baseline levels are indicated by red dotted lines. The frequency of spontaneous Ca 2+ spikes depended on the ZT, which was highest in the middle of the night (ZT18) in PG cells in the CNS–RG complex. ( b ) The Ca 2+ spiking frequencies in PG cells were determined using FFT analysis. In untreated CNS–RG complexes, the wide-band frequency power was higher at ZT18 than at ZT6. The overall frequency power and day–night differences were diminished in CNS–RG complexes cultured with TTX and nimodipine (+TTX/Nim) and in isolated RG cultures. * P <0.05, ** P <0.01 significantly larger than the corresponding ZT6 groups, repeated one-way ANOVA followed by a Duncan's multiple range test. ( c ) The baseline [Ca 2+ ] c levels in PG cells exhibited day–night variations. The highest baseline values were found at ZT6 in untreated CNS–RG complex cultures (control) and CNS–RG complexes cultured with TTX/Nim. The peak baseline value was shifted to ZT18 in isolated RG cultures. * P <0.05, ** P <0.01, one-way ANOVA followed by a Duncan's multiple range test. Full size image In general, a sedative state of [Ca 2+ ] c follows a Ca 2+ spike in endocrine cells. Eventually, baseline [Ca 2+ ] c estimated in PG cells in CNS–RG complex cultures exhibited reversed day–night variations, with the highest [Ca 2+ ] c occurring at ZT6 ( P <0.01 compared with ZT0, number of cells = 130 in 6 organs, one way ANOVA followed by a Duncan's multiple range test; Fig. 7a,c ). In addition, the endogenous clock also drives rhythmic baseline [Ca 2+ ] c in PG cells, because the day–night variations remained visible, with a peak shift from ZT6 to ZT18 in PG cells in the isolated RG ( P <0.01 compared with ZT0, number of cells = 144 in 5 organs, one way ANOVA followed by a Duncan's multiple range test; Fig. 7c ). The intrinsic [Ca 2+ ] c rhythms in PG cells, however, coincided with little Ca 2+ spikes and the amplitudes of circadian variations in baseline [Ca 2+ ] c in PG cells of the isolated RG were smaller than those reported previously for plants [29] and suprachiasmatic nucleus neurons [30] . The present study demonstrates that per -transcriptional rhythms in individual PG cells were autonomous and synchronous, but highly dependent on photoreception in the CNS and efferents from the CNS. Consistently, PER-ir rhythms in PG cells were evident only when they were cultured in the CNS–RG complex under LD cycles. On the other hand, TIM-ir rhythms in PG cells were detected regardless of the CNS. To our knowledge, this is the first report visualizing peripheral cell oscillations with or without the influence of the CNS in an organ culture model and differential PER/TIM oscillations in particular culturing conditions. Furthermore, the present study revealed the spontaneous Ca 2+ spiking activities in PG cells, which were reduced by light exposure to the brain, not to the RG. Ablation of the CNS significantly reduced Ca 2+ spiking frequency in PG cells, and thus PG cells may receive excitatory inputs from the CNS. Rapid reduction of Ca 2+ spiking frequency in PG cells by light exposure to the brain, however, demonstrated that photic signals might be transmitted to PG cells via inhibitory efferent(s). On the basis of these findings, we propose cellular consequences underlying endocrine oscillators and Drosophila eclosion rhythms. The present study demonstrated that the amplitude and photo-entrainability of PG cell per-luc oscillations are highly dependent on the CNS. Interestingly, the result is different from what Liu et al . reported for mammalian fibroblasts [20] , because each PG cell per-luc rhythm was synchronized regardless of the synaptic inputs, whereas the amplitude of per-luc rhythms largely depended on the preceding exposure of the brain to light. Predominant post-translational rhythms (that is, PER-ir levels and Ca 2+ spiking rhythms) in PG cells were also CNS-dependent, suggesting that intrinsic small amplitude per- transcriptional rhythms in PG cells were insufficient to produce robust cellular physiological rhythms within these cells. Significant CNS dependence for photic influence on PG cell rhythms may be inconsistent with the standard concepts of peripheral clocks in flies, because PER-ir and per-luc rhythms in Malpighian tubules synchronize to LD cycles via CRY-dependent mechanisms within the tissues, independent of the CNS [17] , [31] , [32] . Notably, it has been shown that LD entrainment of nuclear PER-ir rhythms is sustained in PG cells in CNS–RG complexes cultured with medium containing 0.3 μM TTX [4] , suggesting CNS-independent PG cell oscillations. The present results, however, demonstrate that circadian rhythms in nuclear PER-ir, if any, were below the detection limits of our curve-fitting analyses in PG cells isolated from the CNS regardless of the lighting schedule. Also, treatment with TTX and nimodipine or physical disconnection of the CNS blocked light-induced amplification of per-luc rhythms in PG cells in CNS–RG complex cultures, suggesting CNS-dependent photoreception and its influence on the circadian oscillations in PG cells. Two explanations may answer the discrepancy between the previous study [4] and ours. First, the previous study did not include less than 60% immunofluorescent signals to estimate PER-ir rhythms [4] and thus, the analytical threshold may underestimate the effect of TTX on PG cell rhythms. Second, TTX may have incompletely blocked CNS influences in the previous study [4] . Indeed, we observed additional effects of Ca 2+ channel blockers on the Ca 2+ spiking activity of PG cells under continuous TTX treatment, although the TTX treatment acutely abolished blue light-induced reduction in Ca 2+ spiking frequencies in PG cells in the present study. It has recently been shown that a subclass of LNs, large ventral LNs in adult flies, exhibit light-dependent action potential firing patterns, with photosensitivity largely dependent on CRY [33] . Therefore, it is likely that photoreception in these central pacemaker neurons substantially strengthen PG cell rhythms. Indeed, light-to-dark rebound amplification of per-luc oscillations in PG cells was blocked in the presence of TTX/nimodipine, in isolated RG or in cry b flies, suggesting that such light-dependent neuronal activity and synaptic signal transduction to PG cells may amplify per- transcriptional oscillations in PG cells. In addition to the significant CNS dependence of per -transcriptional/translational rhythms in PG cells, robust oscillations in nuclear TIM-ir were detected both under LD and DD conditions, regardless of the presence or absence of the CNS. Furthermore, the presence of sustained TIM-ir rhythms even in isolated cry b RG cultures suggests that intrinsic clock mechanisms may generate TIM-ir rhythms. Conversely, immediate synchrony of TIM-ir rhythms to reversed LD cycles in isolated cultures strongly suggests dissociable oscillatory profiles between per and tim in PG cells. This observation was not surprising, because TIM has more direct interaction with and is degraded by CRY following photoreceptions [34] . A prior report also demonstrated dissociation between PER-/TIM-ir rhythms in PG cells under DD [5] . It is important to note, however, that prior results indicating ablation of TIM-ir rhythms under DD in PDF-null mutant ( pdf 01 ) flies [5] are inconsistent with the present results, which indicate CNS-independent TIM-ir rhythms. This discrepancy may simply be due to the number of samples used for these analyses. More importantly, the present results demonstrate that intrinsic TIM oscillations alone could not drive apparent per -transcriptional/translational rhythms and Ca 2+ spiking rhythms in PG cells. Together with prior results showing arrhythmic eclosion under DD by tim over-expression in PG cells [5] , we suggest that coordination of dissociable clock gears may be needed for physiological rhythm generation in this endocrine oscillator. The present study revealed the presence of spontaneous Ca 2+ spikes in PG cells, with peak frequency in the middle of the night and lowest at the onset of light. Also, the present study demonstrates that brief exposure of the CNS to blue light inhibited Ca 2+ spiking activity in PG cells, and that TTX or cry b mutation blocked this effect. This suggests that physiological outputs from PG cell oscillators are under the strong influence of CRY-dependent photoreception in the brain and synaptic inputs to PG cells. Because release of ecdysteroids from PG cells depends on intracellular Ca 2+ signalling [6] , [7] , the lights-on signal would reduce rhythmic ecdysteroid release from PG cells and trigger the endocrine cascade underlying eclosion [8] . This hypothesis is consistent with Drosophila eclosion rhythms, which are known to peak at dawn [35] . Under DD conditions or without CNS influences, PG cell oscillations as per-luc , nuclear PER-ir, and Ca 2+ spiking frequencies were rapidly degraded. These results are consistent with the rapid degradation of circadian ecdysteroid release rhythms under DD reported in Rhodnius prolixus [36] . It is possible that the rapid reduction in PG cell activity under DD opens a temporal gate for eclosion, but the damping PG cell oscillators may not be strong enough to drive robust eclosion rhythms under DD. Thus, additional clock mechanisms may be required to explain circadian eclosion rhythms under DD. It has been shown that LNs project to neurosecretory cells that release eclosion hormone [37] and the other pacemaker neurons, the dorsal neurons, project to cells that release crustacean cardioactive peptide [38] , both of which regulate eclosion downstream from ecdysteroid in the eclosion pathway. This, together with the present data showing that pupal LN oscillations in PER-/TIM-ir levels were robust under DD, suggests that the timing of eclosion is supported via this neuronal pacemaker pathway under DD. Consistent with this, arrhythmic eclosion under DD has been previously observed in LN-ablated or pdf 01 flies [5] . The passive nature of PG cell rhythms in per transcription, nuclear PER expression, and physiological output levels raises the question of the physiological implications of the intrinsic rhythms in PG cells. Overexpression of tim in PG cells results in arrhythmic eclosion patterns [5] , suggesting that PG cell oscillations do have a role regardless of the LNs. Under in vivo conditions, PG cells may receive more diverse signals (for example, temperature cues) to coordinate various zeitgebers, which we did not address in the present study. Thus, the present results do not rule out a possible role of the intrinsic PG cell oscillations in the formation of eclosion rhythms at the system level. In conclusion, we examined the influence of CNS inputs on PG cellular circadian rhythms by monitoring circadian rhythms in per transcription, nuclear PER/TIM expressions, and [Ca 2+ ] c oscillations in PG cells in the CNS–RG complex or isolated RG cultures. The present results demonstrate that circadian rhythms in per transcription in PG cells were self-sustaining and primarily phase-coupled, even in isolated RG cultures. On the other hand, the amplitude of per transcription was largely dependent on prior photic input to PG cells via the CNS. Because photic input via the CNS also amplified the circadian Ca 2+ spiking rhythms, the amplitude of oscillations in both per transcriptions and physiological processes in PG cells seems to depend on neural input. Intracellular Ca 2+ is a potent regulator of diverse physiological processes, including ecdysteroid release, thus the observed oscillatory profiles of PG cells likely contributes to rhythmic ecdysteroid release and eclosion under natural light conditions. Following ablation of photic and synaptic inputs, however, per -transcriptional rhythms and Ca 2+ spiking rhythms were both significantly reduced in PG cells. This reduction may result in a reduction of ecdysteroid release, which then may allow the process of eclosion to proceed; however, the reduced rhythms were not likely to be strong enough to drive rhythmic eclosion independently. Under these circumstances, other circadian pacemakers (possibly neural) may support rhythmic eclosion. Such a synergistic multiple pacemaker system may guarantee the precise timing of eclosion, which is critical for the survival of holometabolous insects. Fly stocks The tim-gal4 , Pdf-gal4 and UAS-GFPll S65T (each on the third chromosome) lines were kindly provided by Dr Daisuke Yamamoto (Tohoku University, Japan). The per-luc (second chromosome) and cry b (third chromosome) lines were kindly provided by Dr Jeffery C. Hall (Brandeis University, MA, USA). The tim-gal4 and UAS-YC2.1-82 (each on the second chromosome) lines were supplied from the Bloomington stock center (Indiana University, IN, USA). All lines were raised on corn meal-molasses-yeast media at 25±1 °C under 12:12-h LD cycle conditions. RG cultures Prepupae 1–3 h after pupariation were selected and dissected during the first 2 h after lights-on. The CNS–RG or isolated RG were dissected in a buffered salt solution containing (mM) 0.5 CaCl 2 , 21.5 KCl, 3.3 KH 2 PO 4 , 15 MgSO 4 , 36 NaCl, 4.8 NaHCO 3 , 4.9 NaH 2 PO 4 , 11.1 d-glucose, and 5.3 sucrose, supplemented with 100 units per ml penicillin, 100 μg ml −1 streptomycin, and 0.25 μg ml −1 amphotericin-B. Isolated tissues were placed on a 0.40-μm cell culture insert (BD Falcon, Franklin Lakes, NJ, USA) and cultured at 25±1 °C in Schneider's Drosophila medium (Invitrogen, Carlsbad, CA, USA) supplemented with 20% (v/v) heat-inactivated fetal bovine serum, 500 ng ml −1 insulin, 100 units per ml penicillin, 100 μg ml −1 streptomycin, and 2.5 μg ml −1 amphotericin-B. Cultures were incubated in a temperature- and humidity-controllable chamber in which a 13-W fluorescent bulb (120–130 lux) was used to produce 12-h:12-h LD cycles. The culture medium was exchanged every 48–60 h. Anti-PER and TIM immunocytochemistry A total of 419 cultured tissues were fixed at different time points using 4% (w/v) paraformaldehyde in PBS for 20 min at room temperature. After fixation, these tissues were blocked in PBS with 10% (v/v) normal donkey serum (Jackson ImmunoResearch, West Grove, PA, USA) and 0.2% (v/v) TritonX-100 (Sigma-Aldrich, St Louis, MO, USA) overnight at 4 °C. These samples were then incubated in 1:1,000 affinity-purified rabbit polyclonal antibody to Drosophila period clock protein (anti-Drosophila PER; Chemicon, Temecula, CA, USA) or in 1:5,000 affinity-purified guinea pig polyclonal antibody to Drosophila TIM [39] (kindly donated by Dr Jaga Giebultowicz, Oregon State University, OR, USA) for 3–4 days at 4 °C. Following five 10-min rinses in PBS, samples were incubated with 1:200 Cy3-conjugated donkey anti-rabbit IgG or with 1:200 Cy5-conjugated anti-guinea pig IgG (Jackson ImmunoResearch) for 48 h at 4 °C. Following five 10-min rinses in PBS, the samples were mounted in Vectashield mounting medium (Vector Laboratories, Burlingame, CA, USA) containing 4',6-diamidino-2-phenylindole. Immunofluorescence images were viewed using a confocal imaging system equipped with an inverted microscope, UPLSAPO 20×NA0.75 objective, and argon/helium neon lasers (Fluoview 1000, Olympus, Tokyo, Japan). Scanning parameters were unified across specimens. Optical intensity was analysed using Adobe PhotoShop CS software (Adobe System, San Jose, CA, USA). PG cells and CA cells were differentiated according to the size of their nuclei: PG cell nuclei were larger than 10 μm and CA cell nuclei were smaller than 7–8 μm. On the basis of this, nuclear PER/TIM levels were calculated for each cell type. The LNs were identified using green fluorescent protein (GFP) fluorescence in Pdf-gal4 / UAS-GFPll S65T flies. The boundaries of the nuclei of LNs were defined in the GFP image and superimposed on the PER/TIM image, and then the average intensity of nuclear regions was calculated. Bioluminescence imaging The CNS–RG complex or isolated RG from per-luc/tim-gal4 ; UAS-GFPll S65T/+ prepupae were cultured on 0.40 μm cell culture inserts (Millicell-CM, Millipore, Billerica, MA, USA) under LD cycle conditions for 36–48 h before recording. Normal Schneider's medium was switched to a medium supplemented with 1 mM beetle luciferin (Promega, Madison, WI, USA) for 1–2 h before recording. Cultures were then incubated in a temperature-controlled (26.5±0.5 °C) custom-built chamber attached to an inverted microscope stage (TE-2000s, Nikon, Tokyo, Japan) by a three-dimensional piezo motor-driven manipulator (Luigs & Neumann, Ratingen, Germany). The bioluminescence images were viewed using a ×20 objective lens (PlanAPO VC20×NA0.75, Nikon) and collected with a 40-min exposure time on a cooled EM-CCD camera (Cascade ll 512B, Photometrics, Tucson, AZ, USA; controlled at −70 °C and 50% EM gain). The images were acquired using digital imaging software (Image Pro-Plus, Media Cybernetics, Bethesda, MD, USA). During the subjective daytime, z -plane focus was adjusted using the motor-driven manipulator under CCD monitoring of the GFP fluorescence image. For this adjustment, bioluminescence imaging was paused and the sample was exposed to a dim blue light (480±10 nm) for 2–10 s using an LED bulb. The intensity of fluorescence was optically invisible but sufficient for detection with the EM-CCD. Individual PG cells in the GFP image were used to estimate the bioluminescence signals located intracellularly. Calcium imaging The CNS–RG complex or isolated RG from tim-gal4 driven UAS-YC2.1-82 prepupae were cultured on 0.40 μm cell culture inserts (Millicell-CM) under LD cycle conditions for 48 h before recording. For short-term Ca 2+ imaging, cultures were gently removed from a filter cup and transferred to the circulating microscope chamber by which buffered-saline solutions similar to the composition of Schneider's medium containing (mM) 5.4 CaCl 2 , 21.5 KCl, 15 MgCl 2 , 36 NaCl, 11.1 d-glucose, 8.3 sucrose, 10 HEPES were perfused at a flow rate of 2.7 ml min −1 . Fluorescence images were observed using an upright microscope (Axioskop, Carl Zeiss, Oberkochen, Germany) with a water-immersion objective lens (Achroplan 40×/0.75, Carl Zeiss). A double-view emission beam splitter (A4313, Hamamatsu Photonics, Shizuoka, Japan) was used to direct two wavelengths simultaneously to a cooled CCD camera (CoolSNAP-Fx, Photometrics). The optical filter sets used were described previously [30] . Recordings and imaging analysis were performed using Metafluor 6.2 software (Universal Imaging Corporation, Buckinghamshire, UK). Excitation light was provided through a liquid light guide from a 175-W Xe lamp (Lambda-LS, Shutter Instrument, Novato, CA, USA) and the exposure time (600 ms every 6-s sampling) was controlled using an electric shutter installed in the lamp. The recording was performed at 24±1 °C. TTX (Wako Pure Chemical Industries, Osaka, Japan), BayK8644 (Sigma-Aldrich), or nimodipine (Sigma-Aldrich) were applied by switching the perfusate. The BayK8644 and nimodipine were dissolved in dimethyl sulfoxide and diluted with buffered-saline solution at a final dimethyl sulfoxide concentration at 0.1% (v/v). Cerebral light stimulation was conducted using a micro-lens attached via an optical fibre (Fiber Tech, Tokyo, Japan) to a deuterium-halogen light source (D2H, World Precision Instruments, Sarasota, FL, USA). Imaging with low-intensity excitations were conducted as above with an EM-CCD camera (Cascade 1k, Photometrics) and an LED bulb (Luxeon-Cool White, Philips Lumileds Lighting, San Jose, CA, USA) instead of a 175-W Xe lamp. For long-term cytosolic Ca 2+ imaging, cultured tissues were monitored for 16 min at 4 different time points (ZT0, 6, 12 and 18) at 24±1 °C under LD cycle conditions. This experimental schedule normalizes gradual damping of spiking activity during 2 consecutive days of recording. Cameleon fluorescence was observed using an upright microscope (ECLIPSE E600, Nikon) with an objective lens (PlanFluor 20×/0.50, Nikon), a mercury short arc lamp (100 W), an excitation filter (435.8 nm DF10, Omega Optical, Brattleboro, VT, USA), an excitation neutral density filter (ND.16), and a dichroic mirror (455SPECIAL C68235, CHROMA, Bellows Falls, VT, USA). The two emission bandpass filters (480DF30 and 535DF25, Omega Optical) were switched using a filter changer wheel (M4312, Hamamatsu Photonics), and the image pairs were collected using a cooled CCD camera (C4880-80, Hamamatsu Photonics). The samples were exposed to the excitation light for 500 ms every 15 s through an electromagnetic shutter (Nidec Copal Electronics, Tokyo, Japan) set in front of the lamp housing. The shutter, filter changer wheel, and image acquisition were regulated using Argus-HiSCA imaging software (Hamamatsu Photonics) installed on a computer. Statistical analysis Means were calculated with standard errors. Nuclear PER and TIM levels from several representative samples were analysed using a regression sine curve fitted with 95% confident levels using SigmaPlot ver 7.0 software (IBM SPSS Statistics, Armonk, NY, USA). The spike frequencies of Ca 2+ oscillations were analysed via FFTs at a frequency range of 0.003–0.03 Hz. Ca 2+ spike frequencies before and after the light exposure were compared using a two-tailed paired t -test. Ca 2+ spike frequencies and baseline [Ca 2+ ] c levels at different ZTs were compared using one way analysis of variance (ANOVA) followed by a Duncan's multiple range test. How to cite this article: Morioka, E. et al . Neuronal influence on peripheral circadian oscillators in pupal Drosophila prothoracic glands. Nat. Commun. 3:909 doi: 10.1038/ncomms1922 (2012).